Creation of skyrmions and antiskyrmions by local heating Heating a system usually increases entropy and destroys order. However, there are also cases where heating gives a system the energy to overcome the potential barrier to reach a state with a nontrivial ordered pattern. Whether heating can manipulate the topological nature of the system is especially important. Here, we theoretically show by microsimulation that local heating can create topological magnetic textures, skyrmions, in a ferromagnetic background of chiral magnets and dipolar magnets. The resulting states depend sharply on intensity and spot size of heating, as well as the interaction to stabilize the skyrmions. Typically, the creation process is completed within 0.1 ns and 10 nm at the shortest time and smallest size, and these values can be longer and larger according to the choice of system. This finding will lead to the creation of skyrmions at will, which constitutes an important step towards their application to memory devices. Thermal agitation plays a crucial role in various fields in physics. Usually, it acts against the coherence and reduces the lifetime of quasiparticles. For example, in magnets, magnons decay with a lifetime that decreases with increasing temperature. However, sometimes, the quasiparticles in magnets can have a long lifetime because of the topology. Namely, when they are characterized by a topological index, which cannot change by the continuous deformation of the magnetic configuration, topological protection makes the lifetime much longer than that for topologically trivial particles. A skyrmion in chiral and dipolar magnets [1] , [2] , [3] , [4] , [5] —a swirling magnetic texture pointing in all directions—is a representative example of this topological particle [6] . In two-dimensional chiral magnets, the Dzyaloshinskii–Moriya (DM) [7] , [8] interaction is allowed and this naturally induces a spiral magnetic structure. As the external magnetic field increases, the ground state changes from a single spiral to a skyrmion crystal and, eventually, to a ferromagnetic state. Dipolar interaction also prefers a nonuniform spiral magnetic configuration to reduce the magnetic field energy, and a similar phase diagram has been obtained in dipolar magnets of finite thickness [9] . The phase transitions are first order, and hence, the metastability of each state persists beyond the phase transition point. The crucial difference between the chiral and dipolar magnets, however, is the presence of the helicity degree of freedom in the latter case as described below [10] . The skyrmion structure in two-dimension is described by where n r is the direction of the magnetic moment at r =( r cos φ , r sin φ ), and the n z axis is taken to be perpendicular to the n x n y plane by the right-hand rule. Here m and φ 0 define the vorticity and the helicity, respectively. The topological skyrmion number N sk is defined as the wrapping number, that is, When we consider a skyrmion in a ferromagnetic background with magnetic moments pointing in the + n z direction (that is, θ r changes smoothly and monotonically from π to 0 for r =0→∞), N sk =− m , independent of the helicity φ 0 . In chiral magnets, the sign of the DM interaction determines the helicity, for example, either φ 0 = π /2 or − π /2, whereas these two structures have the same energy in dipolar magnets. This fact enables richer skyrmion structures in the latter case compared with the former case [11] . The equilibrium properties of skyrmions as well as the current-driven dynamics of skyrmions have been recently studied intensively [12] , [13] , [14] , [15] , [16] , [17] , [18] . Time-dependent nonequilibrium dynamics is an issue of great interest; however, the experimental approach has been rather limited: A Lorentz microscope can map the in-plane components of the magnetization, but the time resolution is of the order of a second, and one cannot follow the rapid dynamics [4] . Small-angle neutron scattering gives information in momentum space and is good at detecting the crystal state of skyrmions, but real space-time information is limited [2] . Among these methods, optical methods [19] , [20] offer powerful tools to excite the system to change the magnetic configuration within a very short time and Faraday rotation spectroscopy enables magnetic-structure detection. However, the latter technique is sensitive only to the out-of-plane component of the magnetic moments, and hence, it cannot be used to determine the topological nature of the resultant magnetic textures. Also the real-time dynamics of the creation process is not explored. Therefore, theoretical studies of the real-time nonequilibrium dynamics induced by local heating are highly desirable to develop the design principle of optical manipulation of the magnetic textures as well as to understand the existing experiments. From an application viewpoint, solid-state phase control by local heating is widely used for memory devices (for example, laser heating has been used for recordable and/or rewritable magneto-optical discs, compact discs, digital versatile discs, Blu-ray discs and so on (see Fig. 1 )). For higher density memory devices, the focused spot size of the laser irradiation continues to be reduced, currently reaching a diameter of ~0.58 μm for Blu-ray discs [21] . Studies of local heating beyond the optical diffraction limit are in progress, and an ~10-nm scale control has already been achieved by using near-field techniques in nano-optics [22] . Local heating using atomic force microscope techniques [23] also has considerable potential for nanoscale control. These techniques are useful to create and annihilate skyrmions at will as shown below. 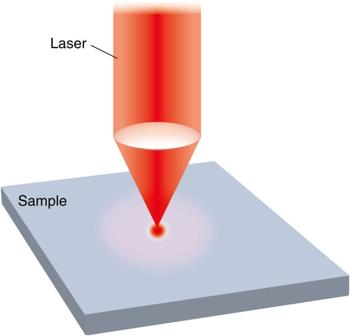Figure 1: Schematic figure of local heating by laser irradiation.  Figure 1: Schematic figure of local heating by laser irradiation. Full size image Numerical simulation In the present paper, we study the creation and annihilation of the skyrmion by local heating by solving the stochastic Landau–Lifshitz–Gilbert equation given by where is the Hamiltonian and the Gaussian noise field h T ( r ) ( t )=( h T ( r ), x ( t ), h T ( r ), y ( t ), h T ( r ), z ( t )) with the statistical properties ‹ h T ( r ), ν ( t )›=0 and ‹ h T ( r ), μ ( t ) h T ( r ′), ν ( t ′)›=2 k B T ( r ) αδ μν δ ( r – r ′) δ ( t – t ′) ( μ , ν = x , y , z ) is introduced to examine the effect of local heating by a spatially dependent temperature T ( r ) on the Langevin dynamics of the system. To solve this equation, we use the Heun scheme [24] and the random-number generator developed by M. Matsumoto and T. Nishimura ( http://www.math.sci.hiroshima-u.ac.jp/~m-mat/MT/emt.html ) for the Gaussian noise field h T ( r ) ( t ). Skyrmion creation and annihilation in chiral magnet by local heating First, we examine skyrmion creation by local heating in a chiral magnet. The model Hamiltonian for the chiral magnet defined on a two-dimensional square lattice is given by where e x and e y are the unit vectors in the x and y directions, respectively, and we take the lattice constant a as the unit of length. 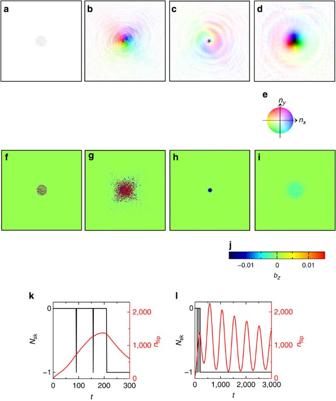Figure 2: Skyrmion creation by heat. The parameter set {D/J=0.15,h/J=0.015,α=0.01} is used on anL=300 × 300 square lattice system with periodic boundary condition. Hereafter, we takeJas the unit of energy and the lattice constantaas the unit of length. Correspondingly, 1/(γJ) is the unit of time. If we assumeγ=gsμB/ℏ(gs: electron sping-factor,μB: Bohr magneton) andJ=10−3eV, 1/(γJ)=0.7 ps. The initial state is a perfect ferromagnetic state withnz,r=+1. (a–d) The magnetic textures att=1, 200, 350 and 570, respectively. The colour map (e) specifies the magnetic moment. The brightness of the colour represents thezcomponent of the magnetic moment; that is, the bright (dark) colour is for positive (negative)nz, and hence white (black) corresponds tonz=+1 (nz=−1). During 0≤t≤theating=200, local heating corresponding tokBT/J=1.0 is applied at the centre region with radiusR=20. (f–i) The spatial distribution of the solid angle (with a factor 1/2) formed by four magnetic moments on the plaquette,, for the magnetic textures shown ina–d, respectively. The scale forbzis shown inj. (k) Time dependence of skyrmion numberNsk(black with the left scale) andnflip=∑r(1–nz,r)/2 (red with the right scale). (l) The same askbut for 0≤t≤3,000. Figure 2 shows the result for a finite size L =300 × 300 system with periodic boundary condition and the parameter set { D / J =0.15, α =0.01, h / J =0.015}. The nondimensional time is measured in units of 1/( γJ ). A small time increment of 0.01 is used for the numerical time evolution of equation (3). Note that the critical magnetic field h c (refs 25 , 26 ) separating the skyrmion crystal state and the ferromagnetic state in the ground state is h c / J =0.0175 for D / J =0.15. Therefore, the perfect ferromagnetic state, which is the initial state in this simulation, is a metastable state for h / J =0.015. In the initial stage, 0≤ t ≤ t heating =200, local heating corresponding to k B T / J =1.0 is applied at the centre region with radius R =20 in units of a , that is, T ( r )=0 for | r − r c | > R and T ( r )= T for | r − r c | ≤ R , where r c is the centre of Fig. 2a–d , which show representative snapshots of the time evolution of the magnetic structure. We also show the spatial distribution of the solid angle (with a factor 1/2) formed by four magnetic moments on the plaquette, , in Fig. 2f–i for each of Fig. 2a–d . It has been known that b z can be physically interpreted as the emergent magnetic field acting on the conduction electrons coupled to the magnetic moments [27] , [28] , [29] . Note that and its time dependence is shown in Fig. 2k,l by the black line. In the initial stage, 0≤ t ≤ t heating =200, owing to the stochastic force h T ( r ) ( t ) corresponding to the high-temperature k B T = J at | r − r c |≤ R , the magnetic moments are strongly disordered in the central area, as seen in Fig. 2a–b . We define n flip =∑ r (1− n z , r )/2, which gives an estimate for the number of flipped magnetic moments from the ferromagnetic state, and plot it in Fig. 2k,l by red curves. The time dependence in N sk shows some spiky structures for 0≤ t ≤ t heating =200, because the topological skyrmion number is ill-defined for the strongly disordered magnetic structure. For t heating =200< t , the heat is turned off, that is, T ( r )=0 for the whole system, so that the excited system relaxes to a spatially slowly varying magnetic texture. At the same time, the topological skyrmion number N sk becomes well defined. Finally, a skyrmion is created (see Fig. 2c,h,k,l) . Later, the created skyrmion exhibits a breathing motion along with the relaxation dynamics. Consequently, n flip exhibits a damped oscillation, that is, with increasing (decreasing) n flip , the skyrmion is expanding (shrinking; see Fig. 2c,d,h,i and the red curve in Fig. 2l ). Figure 2: Skyrmion creation by heat. The parameter set { D / J =0.15, h / J =0.015, α =0.01} is used on an L =300 × 300 square lattice system with periodic boundary condition. Hereafter, we take J as the unit of energy and the lattice constant a as the unit of length. Correspondingly, 1/( γJ ) is the unit of time. If we assume γ = g s μ B / ℏ ( g s : electron spin g -factor, μ B : Bohr magneton) and J =10 −3 eV, 1/( γJ )=0.7 ps. The initial state is a perfect ferromagnetic state with n z , r =+1. ( a – d ) The magnetic textures at t =1, 200, 350 and 570, respectively. The colour map ( e ) specifies the magnetic moment. The brightness of the colour represents the z component of the magnetic moment; that is, the bright (dark) colour is for positive (negative) n z , and hence white (black) corresponds to n z =+1 ( n z =−1). During 0≤ t ≤ t heating =200, local heating corresponding to k B T / J =1.0 is applied at the centre region with radius R =20. ( f – i ) The spatial distribution of the solid angle (with a factor 1/2) formed by four magnetic moments on the plaquette, , for the magnetic textures shown in a – d , respectively. The scale for b z is shown in j . ( k ) Time dependence of skyrmion number N sk (black with the left scale) and n flip =∑ r (1– n z , r )/2 (red with the right scale). ( l ) The same as k but for 0≤ t ≤3,000. Full size image The skyrmion creation by local heating depends not only on the intensity of heat but also on the heating period t heating . The final result of the magnetic texture calculated by the Langevin dynamics following equation (3) is different every time because of the randomly supplied stochastic force h T ( r ) ( t ) at the initial stage. Therefore, the skyrmion creation sometimes fails even under the same numerical parameters α , k B T , R , t heating and those in the Hamiltonian . At the same time, the probability of skyrmion creation increases for longer t heating . 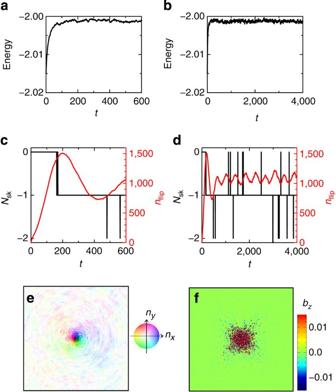Figure 3: Effect of continuous local heating. The parameter set {D/J=0.15,h/J=0.015,α=0.01} is used on anL=300 × 300 square lattice system with periodic boundary condition. The spot of radiusR=20 is heated continuously atkBT/J=1.0. (a) Time dependence of the total energy divided byL. (b) The same asa, but for 0≤t≤4,000. (c) Time dependence ofNsk(black with the left scale) andnflip(red with the right scale). (d) The same asc, but for 0≤t≤4,000. (e) Magnetic texture att=4,000. (f) Spatial distribution ofbzatt=4,000. Figure 3 shows the result where local heating corresponding to k B T / J =1.0 is applied continuously at the centre region with radius R =20. Other numerical conditions are the same as those in Fig. 2 . For the total energy divided by the system size L ( Fig. 3a ), a characteristic saturation time ~1/ α (=100 in units of 1/( γJ ) in this case) is seen. For t ≳ 200, although an oscillation with a small amplitude is seen in the time dependence of n flip (see Fig. 3c,d ), the system almost reaches a steady state; that is, the magnetic texture and spatial distribution of b z are always similar to those of Fig. 3e,f , respectively. We find that, in this numerical study on finite size systems, a period t heating =1,000 is enough for skyrmion creation by local heating, and longer heating does not change the skyrmion-creation efficiency. It is interesting to note that, despite the spiky behaviour of N sk seen in Fig. 3c,d , it takes −1 almost everywhere; that is, the parameter set here gives a favourable condition for skyrmion creation by local heating. In the early stage towards the steady state, we find an overshoot behaviour in the time dependence of n flip at t =200 (see Fig. 3c,d ), which represents a strong local deformation of the magnetic texture from the perfect ferromagnetic state. Figure 3: Effect of continuous local heating. The parameter set { D / J =0.15, h / J =0.015, α =0.01} is used on an L =300 × 300 square lattice system with periodic boundary condition. The spot of radius R =20 is heated continuously at k B T / J =1.0. ( a ) Time dependence of the total energy divided by L . ( b ) The same as a , but for 0≤ t ≤4,000. ( c ) Time dependence of N sk (black with the left scale) and n flip (red with the right scale). ( d ) The same as c , but for 0≤ t ≤4,000. ( e ) Magnetic texture at t =4,000. ( f ) Spatial distribution of b z at t =4,000. 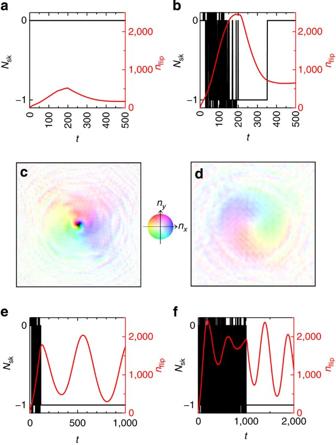Figure 4: Efficiency of skyrmion creation by heating. The parameter set {D/J=0.15,h/J=0.015,α=0.01} is used on anL=300 × 300 square lattice system with periodic boundary condition. The local heating corresponding tokBT/J=0.5 is used foraandkBT/J=1.5 is used forb–d. (a,b) Time dependence ofNsk(black with the left scale) andnflip(red with the right scale). (c,d) The magnetic textures att=300 and 500, respectively, in caseb. The colour map incspecifies the magnetic moment. The results with the numerical conditions inbexcept (e)theating=100 and (f)theating=1,000, respectively. Full size image Figure 4 displays how the skyrmion-creation efficiency depends on the intensity of local heating. The numerical conditions are the same as those in Fig. 2 , except k B T / J =0.5 in Fig. 4a and k B T / J =1.5 in Fig. 4b–d , respectively. In the case of Fig. 4a , the effect of local heating and n flip are not large enough to create the skyrmion and N sk stays always zero. In contrast, strong heating can create the skyrmion but also destroy it, as shown in Fig. 4b–d where k B T / J =1.5. In this case, the heating is stopped at t = t heating =200, where the overshoot reaches almost maximum. For the parameter set used in Fig. 4b , we examine t heating dependence. Figure 4e,f are the cases with t heating =100 and 1,000, respectively. In the former case, the local heating is turned off before the overshoot reaches the maximum. Consequently, n flip at t = t heating , which is the key factor, is smaller than that in the case Fig. 4b , and the created skyrmion is not destroyed. The skyrmion survives also in the case with t heating =1,000 where the local heating is turned off after maximum of the overshoot occurs. This is because the local deformation represented by n flip is not strong enough in comparison to the case in Fig. 4b (In Fig. 4f , n flip at t =1,400 reaches similar value ( n flip =2,400–2,500) at the overshoot stage, but those magnetic textures are completely different from each other, that is, the magnetic texture at t =1,400, after turned off the heating, has a well-defined skyrmion number N sk =−1, whereas N sk is ill-defined during heating. The former magnetic texture is arranged by slowly varying magnetic moments, whereas the magnetic moments are strongly disordered in the latter one. Consequently, turning off of the local heating at the overshoot stage destroys the created skyrmion but not in the case of Fig. 4f ). By changing t heating with 50 increments, we perform the numerical simulation ten times for each t heating . We find the behaviour similar to the case of Fig. 4b for 200≤ t heating ≤250 with 100% probability, that is, the skyrmion is created once but it is destroyed later. For 100 ≤ t heating ≤150 and 350≤ t heating , on the other hand, the created skyrmion by the local heat is not destroyed. Figure 4: Efficiency of skyrmion creation by heating. The parameter set { D / J =0.15, h / J =0.015, α =0.01} is used on an L =300 × 300 square lattice system with periodic boundary condition. The local heating corresponding to k B T / J =0.5 is used for a and k B T / J =1.5 is used for b – d . ( a , b ) Time dependence of N sk (black with the left scale) and n flip (red with the right scale). ( c , d ) The magnetic textures at t =300 and 500, respectively, in case b . The colour map in c specifies the magnetic moment. The results with the numerical conditions in b except ( e ) t heating =100 and ( f ) t heating =1,000, respectively. Full size image We examine the effect of heating on skyrmion creation by changing widely the intensity and spot size of the local heating (In ref. 20 , the laser power dependence in skyrmion, skyrmionium, di-skyrmionium creations is discussed. The detailed discussion on skyrmionium and di-skyrmionium is shown below. Here, we examine the effect of not only the heating power but also the spot size of local heating on the skyrmion creation and annihilation; therefore, our results give a possible way to control the resultant magnetic texture by controlling the spot size and the temperature.). The results are summarized in Fig. 5 in the plane of k B T and R . Owing to the stochastic nature of the Langevin dynamics by equation (3), we examine each point on the R − k B T plot in Fig. 5 at least ten times with several t heating ’s up to 1,000. In the grey region of Fig. 5a , we find single-skyrmion creation by heating. The probability of single-skyrmion creation is highest deep inside the grey region, and it decreases towards the boundaries. The points k B T / J =1.5 and 2.0 with R =20 are in the yellow region, which means that the skyrmion is created once but is destroyed later by the strong heat depending on t heating , as discussed above. For k B T / J =2.0, the skyrmion is destroyed finally for 150≤ t heating ≤200, but it survives for 50≤ t heating ≤100 and 400≤ t heating with 100% probability (For t heating =50, the skyrmionium is found on rare occasion, that is, less than 10% of the attempts.). When we increase the Gilbert damping α with the same k B T and R , we find skyrmion creation without its destruction afterward. These cases are shown in Fig. 5b,c,d , which display the results for α =0.05, 0.1 and 1.0, respectively. Larger damping, however, also brings about different magnetic textures other than the single skyrmion. 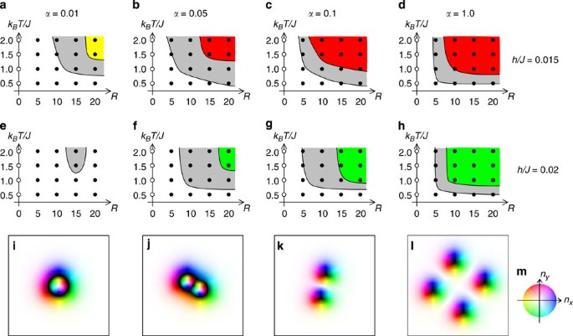Figure 5: Skyrmion creation by heating with various magnitude inαandh/Jon aR–kBTplot. The local heating corresponding toT(r)=T(T(r)=0) for |r–rc| ≤R(|r–rc| >R) is applied with (a)α=0.01, (b)α=0.05, (c)α=0.1 and (d)α=1.0, respectively, andh/J=0.015. Panelse–hare the same asa–d, respectively, but forh/J=0.02. The closed dots indicate the points studied numerically. The coloured areas (grey, yellow, red and green) are guide for eyes to distinguish the efficiency and types of skyrmion production by local heating: In the grey region, we find single-skyrmion creation. In the yellow region, there is range oftheating, where the skyrmion is created once but is destroyed later. In the red region, not only the single-skyrmion but also the magnetic textures shown ini–lare found. In the green region, we find several-skyrmion creation in addition to single-skyrmion creation without the composite magnetic textures likeiandj. The examples of the magnetic textures, (i) single skyrmionium at {α=0.05,R=15,kBT=1.0}, (j) di-skyrmionium at {α=0.05,R=20,kBT=1.0}, (k) two skyrmions at {α=0.1,R=20,kBT=1.5} and (l) four skyrmions at {α=1.0,R=20,kBT=1.0} are shown using the colour map (m), which specifies the magnetic moment. These are the snapshots within the area of 150a× 150a, att=5,000. The similar magnetic textures are also found at other points in the red regions. Figure 5i–l shows examples and is found in the red regions in Fig. 5b–d . The magnetic textures of Fig. 5i,j are called skyrmionium and di-skyrmionium by Finazzi et al. [20] : in the skyrmionium in Fig. 5i , the magnetic moment at the centre r centre is parallel to the z axis, that is, . Along the radial direction from the centre, the magnetic moments wind by 2 π in a manner compatible with the DM interaction. As a result, sites with n z , r =−1 form a ring and divide the system into two regions, that is, inside and outside of the ring. The magnetic moments inside (outside) of the ring wrap the sphere with a solid angle+4 π (−4 π ) and hence N sk =0 in the skyrmionium. In other words, skyrmionium is a composite structure of an antiskyrmion (inside) and a skyrmion (outside). The di-skyrmionium shown in Fig. 5j is composed of two antiskyrmions with N sk =+1 surrounded by the skyrmion structure with N sk =−1. As a result, the di-skyrmionium has N sk =+1. In addition to creation of single skyrmion, skyrmionium and di-skyrmionium, we find several-skyrmion creation, as shown in Fig. 5k,l . Figure 5: Skyrmion creation by heating with various magnitude in α and h / J on a R – k B T plot. The local heating corresponding to T ( r )= T ( T ( r )=0) for | r – r c | ≤ R (| r – r c | > R ) is applied with ( a ) α =0.01, ( b ) α =0.05, ( c ) α =0.1 and ( d ) α =1.0, respectively, and h / J =0.015. Panels e – h are the same as a – d , respectively, but for h / J =0.02. The closed dots indicate the points studied numerically. The coloured areas (grey, yellow, red and green) are guide for eyes to distinguish the efficiency and types of skyrmion production by local heating: In the grey region, we find single-skyrmion creation. In the yellow region, there is range of t heating , where the skyrmion is created once but is destroyed later. In the red region, not only the single-skyrmion but also the magnetic textures shown in i – l are found. In the green region, we find several-skyrmion creation in addition to single-skyrmion creation without the composite magnetic textures like i and j . The examples of the magnetic textures, ( i ) single skyrmionium at { α =0.05, R =15, k B T =1.0}, ( j ) di-skyrmionium at { α =0.05, R =20, k B T =1.0}, ( k ) two skyrmions at { α =0.1, R =20, k B T =1.5} and ( l ) four skyrmions at { α =1.0, R =20, k B T =1.0} are shown using the colour map ( m ), which specifies the magnetic moment. These are the snapshots within the area of 150 a × 150 a , at t =5,000. The similar magnetic textures are also found at other points in the red regions. Full size image We also examine skyrmion creation by heating for h / J =0.02, and the results are summarized in Fig. 5e–h , where the other numerical conditions are the same as those in Fig. 5a–d . In this case, the perfect ferromagnetic state is the ground state. In the green region, we find several-skyrmion creation in addition to single-skyrmion creation, but neither skyrmionium nor di-skyrmionium creation. In Fig. 5e , there are two kinds of phase boundaries. The former is lying at the left end of the grey area and is determined by the threshold strength of heating to create a skyrmion. On the other hand, the right end of the grey area gives a threshold heat to destroy the created skyrmion at the initial stage, that is, at the points k B T =1.5 and 2.0 with R =20 in Fig. 5e , the skyrmion is created once but disappears later with 100% probability because of the strong heat even in the case that the local heating is turned off after maximum of the overshoot occurs, in contrast to case of the yellow region in Fig. 5a . Let us explore the skyrmion nucleation process in more depth. 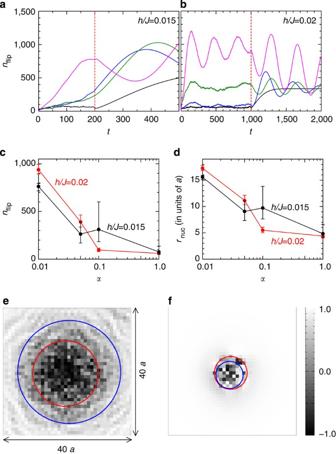Figure 6: Nucleation process of a skymion. (a) Time dependence innflipforh/J=0.015 andtheating=200 (vertical-red-broken-line) atkBT/J=2.0 with (α,R)=(1.0,5), (0.1,5), (0.05,5) and (0.01,10) are shown by black, blue, green and pink curves, respectively. (b) Thet–nflipplot forh/J=0.02 andtheating=1,000 (vertical-red-broken-line) atkBT/J=2.0 with (α,R)=(1.0,5), (0.1,5), (0.05,10) and (0.01,15) are shown by black, blue, green and pink curves, respectively. (c) Theα–nflipplot att=theatingwith (α,R)=(1.0,5), (0.1,5), (0.05,5) and (0.01,10) forh/J=0.015, and (α,R)=(1.0,5), (0.1,5), (0.05,10) and (0.01,15) forh/J=0.02. The average (dots) and the error bars are calculated for ten attempts of the numerical simulation of the Langevin dynamics by equation (3). (d) Theαdependence of the critical radius of the nucleation centre, (a: the lattice constant). (e,f) The spatial distributions ofnz,r(the grey scale is shown inf) in an area of 40a× 40aatt=theating=200 on the black and pink curves in the plota, respectively. The red circles indicate the heating spots. The blue circles centred at the pointwith the radiusrnuc(≈15.7aineand ≈4.1ainf) are also shown. Figure 6 summarizes the nucleation characteristics on the left ends of the grey regions in Fig. 5a–h at k B T / J =2.0. To observe the nucleation process, t heating =200 and 1,000 are taken for h / J =0.015 and 0.02, respectively, because for h / J =0.015 the time-evolution turns into the skyrmion breathing motion stage during the local heating for longer t heating ≥200. Figure 6a,b shows the time dependence of n flip . For smaller α , the skyrmion creation needs larger n flip . In particular, for α =0.01, the heating must be applied at larger sizes, R =10 or 15, whereas R =5 is enough in the cases with α =0.1 and 1.0. In Fig. 6c , we plot the α dependence in n flip at t = t heating , that is, average (dots) and the error bars are calculated for ten attempts of the numerical simulation of the Langevin dynamics by equation (3). Note that the critical R for the skyrmion creation is dependent on α . This critical R value, however, is somehow related but not exactly the size of the critical nucleation centre of the skyrmion formation. On the data in Fig. 6c , we define Figure 6: Nucleation process of a skymion. ( a ) Time dependence in n flip for h / J =0.015 and t heating =200 (vertical-red-broken-line) at k B T / J =2.0 with ( α , R )=(1.0,5), (0.1,5), (0.05,5) and (0.01,10) are shown by black, blue, green and pink curves, respectively. ( b ) The t – n flip plot for h / J =0.02 and t heating =1,000 (vertical-red-broken-line) at k B T / J =2.0 with ( α , R )=(1.0,5), (0.1,5), (0.05,10) and (0.01,15) are shown by black, blue, green and pink curves, respectively. ( c ) The α – n flip plot at t = t heating with ( α , R )=(1.0,5), (0.1,5), (0.05,5) and (0.01,10) for h / J =0.015, and ( α , R )=(1.0,5), (0.1,5), (0.05,10) and (0.01,15) for h / J =0.02. The average (dots) and the error bars are calculated for ten attempts of the numerical simulation of the Langevin dynamics by equation (3). ( d ) The α dependence of the critical radius of the nucleation centre , ( a : the lattice constant). ( e , f ) The spatial distributions of n z , r (the grey scale is shown in f ) in an area of 40 a × 40 a at t = t heating =200 on the black and pink curves in the plot a , respectively. The red circles indicate the heating spots. The blue circles centred at the point with the radius r nuc (≈15.7 a in e and ≈4.1 a in f ) are also shown. Full size image for an estimate for the radius of the skyrmion nucleation centre, and its α dependence is shown in Fig. 6d . Figure 6e,f is the real-space images of the skyrmion nucleation centres corresponding to the points at t = t heating on the black and pink curves in Fig. 6a , respectively. The precession dynamics of the magnetic moments is active for small α ( ≪ 1.0), whereas suppressed for larger damping case. Correspondingly, for α =0.01, the energy flow occurs from inside to outside of the heating spot ( Fig. 6e ), whereas the excitation energy is almost confined at around the heating spot for α =1.0 ( Fig. 6f ). Because of the energy flow, the larger k B T / J and R are needed to create a skyrmion for smaller α =0.01 ( Fig. 6e ) compared with the case of α =1.0 ( Fig. 6f ). In the latter case, the radius r nuc ≅ 4.1 (blue circle) is overestimated as a small number of flipped magnetic moments (the deep-dark pixels in Fig. 6f ) is enough for the skyrmion nucleation. In the overdamped case, the precession of the magnetic moments are strongly suppressed and the system is expected to obey the relaxation dynamics on the adiabatic energy surfaces. Therefore, we analyse below an adiabatic energy profile for a simplified model: Assume a single magnetic moment at the centre r =0 is flipped and the surrounding four moments are twisted accordingly due to the DM interaction (Here we consider the square lattice with lattice constant a . ). This situation is described by the configuration as n r =(−sin φ sin θ r ,cos φ sin θ r ,cos θ r ), at the site r =( r cos φ , r sin φ ) (This corresponds to m =+1 and φ 0 = π /2 in equation (1)). The angle θ r for the neighbouring four magnetic moments is put to be θ a , and the rest of the magnetic moments are treated in the continuum approximation. With these assumptions, the energy E ({ θ r }) estimated from the Hamiltonian equation (4) is given by We employ the variational method to estimate the energy functional E ({ θ r }) with the constraint θ r = a = θ a . The varitational function is chosen to be n z , r =cos θ r =1−2 A exp[−( r / r 0 ) 2 ] [20] , for 0< A <1 and a < r 0 . 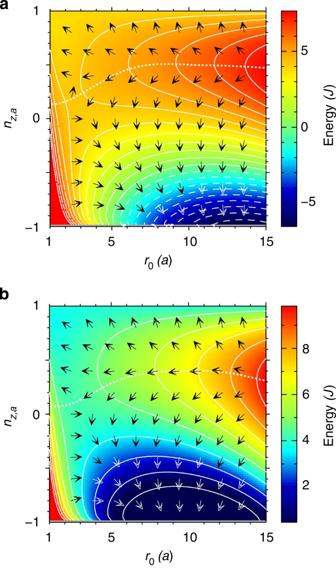Figure 7: Contour map of energyE({θr}) expressed by equation (6) onr0−nz,a(=cosθa) plane. The parameters (a)D/J=0.15 andh/J=0.015 (b)h/J=0.02 are used. The white solid (broken) curves are the equal-energy lines with positive (negative) energy, whereas the arrows represent the gradient of the energy, which specifies the direction to lower the energy. The white dotted curve indicates the separatrix for the two stable points. Figure 7 shows contour map of the energy on the r 0 − n z , a plane for h / J =0.015 and 0.02 with D / J =0.15. The white solid (broken) curves are the equal-energy lines with positive (negative) energy, whereas the arrows represent the gradient of the energy which specifies the direction to lower the energy. The white dotted curve indicates the separatrix for the two stable points, that is, (i) n z , a ≃ +1, r 0 ≃ 1. In this case, the magnetic moment at site 0 is also easily reversed by tiny disturbance, and the system goes back to the ferromagnetic state and (ii) r 0 ≅ 14 for h / J =0.015 and r 0 ≅ 10 for h / J =0.02 with n z , a ≅ −1 corresponding to the skyrmion formation. This implies that only the one reversed magnetic moment surrounded by the neighbouring ones with n z , a ≲ 0 is enough to create a skyrmion in the ferromagnetic background. This describes the skyrmion nucleation in the overdamped case in Fig. 6f reasonably well. For smaller α , on the other hand, due to the nonequilibrium nature of the real-time dynamics of the magnetic moments, the mutual precession of the magnetic moments tends to recover the ferromagnetic state. In other words, although the chiral magnet has an instability of the skyrmion-nucleation discussed above, a mass of reversed magnetic moments at the region with a several hundreds of sites are required to achieve the skyrmion-creation for small α . Figure 7: Contour map of energy E ({ θ r }) expressed by equation (6) on r 0 − n z , a (=cos θ a ) plane. The parameters ( a ) D / J =0.15 and h / J =0.015 ( b ) h / J =0.02 are used. The white solid (broken) curves are the equal-energy lines with positive (negative) energy, whereas the arrows represent the gradient of the energy, which specifies the direction to lower the energy. The white dotted curve indicates the separatrix for the two stable points. Full size image The phase diagram shown in Fig. 5 is useful not only for skyrmion creation but also for skyrmion annihilation. As discussed above, at the points k B T / J =1.5 and 2.0 with R =20 in Fig. 5a,e , the heating is too strong for the skyrmion. In other words, strong heating can eliminate the skyrmion. 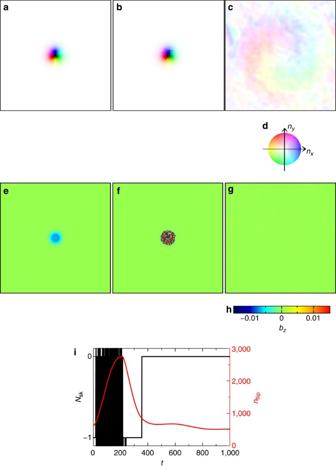Figure 8: Skyrmion annihilation by heating. The initial state is the stabilized single-skyrmion configuration. The parameter set {D/J=0.15,h/J=0.015,α=0.01,R=20,kBT/J=2.0,theating=200} is used on anL=300 × 300 square lattice system with periodic boundary condition. (a–c) The magnetic textures att=0, 1 and 1,000, respectively. The colour map (d) specifies the magnetic moment. (e–g) The spatial distribution ofbzatt=0, 1 and 1,000, respectively. The scale forbzis shown inh. (i) Time dependence ofNsk(black with the left scale) andnflip(red with the right scale). Figure 8 shows the process of skyrmion annihilation. The parameter set is the same as that for the point { R =20, k B T / J =2.0} in Fig. 5a . First, we prepare the stabilized single-skyrmion state (see Fig. 8a ) for the initial state. Heat is applied during 0< t < t heating =200 and later the heating is turned off. As seen in the spatial distribution of b z ( Fig. 8f ) and n flip (red curve in Fig. 8i ), the effect of heating immediately appears. At t =360, the skyrmion number N sk becomes zero (see black line in Fig. 8i ); that is, skyrmion annihilation is completed. In the same way, we examined skyrmion annihilation at the points k B T / J =1.5 and 2.0 with R =20 in Fig. 5a,e . The efficiency of skyrmion annihilation is 100%, at least in our numerical study. At the points in the grey region of the phase diagram, local heating does not eliminate the stabilized single skyrmion. Figure 8: Skyrmion annihilation by heating. The initial state is the stabilized single-skyrmion configuration. The parameter set { D / J =0.15, h / J =0.015, α =0.01, R =20, k B T / J =2.0, t heating =200} is used on an L =300 × 300 square lattice system with periodic boundary condition. ( a – c ) The magnetic textures at t =0, 1 and 1,000, respectively. The colour map ( d ) specifies the magnetic moment. ( e – g ) The spatial distribution of b z at t =0, 1 and 1,000, respectively. The scale for b z is shown in h . ( i ) Time dependence of N sk (black with the left scale) and n flip (red with the right scale). Full size image Skyrmion and antiskyrmion creation in dipolar magnet by local heating Next, we examine skyrmion creation by heating in a dipolar magnet. The model Hamiltonian on a two-dimensional square lattice is given by Using this Hamiltonian, we solve the stochastic Landau–Lifshitz–Gilbert equation equation (3). 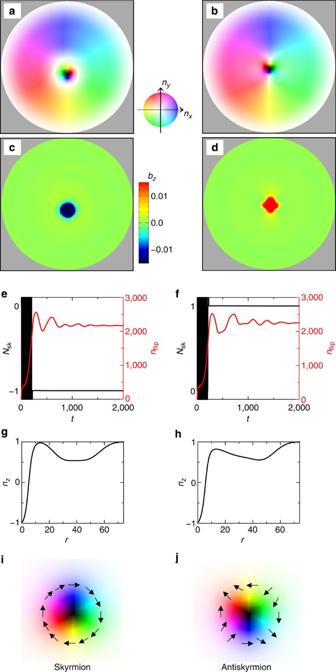Figure 9: Skyrmion (a) and antiskyrmion (b) creation by heating in a dipolar magnet. The system is the disc with a diameter of 150 lattice spacings (17,663 sites are involved) in free boundary condition. The parameter set {theating=200,Idip/J=0.094,A/J=0.6,h/J=0.04,α=0.1,kBT=2.0,R=15,L=17,663} is used. The colour map inaspecifies the magnetic moment. These figures are the snapshots observed att=2,000. (c,d) The spatial distribution ofbzforaandb, respectively. The scale forbzis shown inc. (e,f) The time dependence ofNsk(black with left scale) andnflip(red with right scale) foraandb, respectively. (g,h) The profiles ofnz,rof the magnetic textures foraandb, respectively, withr(r=rex) from the centre of the magnetic textures. Schematic representation of (i) skyrmion (Nsk=−1) and (j) antiskyrmion (Nsk=+1). The arrows indicate the in-plane component of the magnetic moments. Figure 9 shows the result for a disc-shaped system, in which the disc diameter is 150 lattice spacings and the number of sites in the disc is L =17,663. A parameter set { I dip / J =0.094, A / J =0.6, h / J =0.04, α =0.1, k B T =2.0, R =15} is used. Similar to the calculation for Fig. 2 , the initial state is a perfect ferromagnetic state with n z , r =+1, local heating corresponding to k B T / J =2.0 is applied at the centre region with radius R =15 during 0≤ t ≤ t heating =200, and T ( r )=0 for 200< t . We find both skyrmion ( N sk =−1) and antiskyrmion ( N sk =+1) final states (see Fig. 9 ) depending on the random-number generation. Note that the respective spatial structures of n z , r in Fig. 9g,h are similar to each other, so that information on the out-of-plane component of the magnetic moments is insufficient and observation of their in-plane component is necessary to determine the topological nature of the magnetic texture. This is a characteristic of dipolar magnets; that is, they have a large number of metastable states. The result depends on the random numbers generated to solve equation (3), so that a skyrmion or antiskyrmion with different helicity appears stochastically, and sometimes no skyrmion creation occurs. Figure 9: Skyrmion (a) and antiskyrmion (b) creation by heating in a dipolar magnet. The system is the disc with a diameter of 150 lattice spacings (17,663 sites are involved) in free boundary condition. The parameter set { t heating =200, I dip / J =0.094, A / J =0.6, h / J =0.04, α =0.1, k B T =2.0, R =15, L =17,663} is used. The colour map in a specifies the magnetic moment. These figures are the snapshots observed at t =2,000. ( c , d ) The spatial distribution of b z for a and b , respectively. The scale for b z is shown in c . ( e , f ) The time dependence of N sk (black with left scale) and n flip (red with right scale) for a and b , respectively. ( g , h ) The profiles of n z , r of the magnetic textures for a and b , respectively, with r ( r = r e x ) from the centre of the magnetic textures. Schematic representation of ( i ) skyrmion ( N sk =−1) and ( j ) antiskyrmion ( N sk =+1). The arrows indicate the in-plane component of the magnetic moments. Full size image Last, we discuss the relevance of the present results to the experiments. In refs 19 , 20 , submicron-scale magnetization reversal is induced by optical pulse irradiation in a TbFeCo thin film with a spot size ~1 μm. In this system, the magnetic bubble is stabilized by the dipolar interaction, and hence, its size is relatively large (~500 nm). The laser spot size is of the same order. This is semiquantitatively consistent with our simulation as follows. From the Curie temperature ~500 K, the exchange coupling is estimated to be J =10 meV. Therefore, the unit of time 1/( γJ )=0.07 ps, so that the result of Fig. 9 corresponds to the case with a heating period t heating =200 × 1/( γJ )=14 ps. The typical local-temperature increase induced by laser irradiation has been estimated in TbFeCo thin film as ~800 K (~1.6 times larger than T c ) [30] . This value is also consistent with k B T / J ≲ 2.0 used in the present numerical study. How to cite this article : Koshibae, W. and Nagaosa, N. Creation of skyrmions and antiskyrmions by local heating. Nat. Commun. 5:5148 doi: 10.1038/ncomms6148 (2014).